Structural insights of human mitofusin-2 into mitochondrial fusion and CMT2A onset Mitofusin-2 (MFN2) is a dynamin-like GTPase that plays a central role in regulating mitochondrial fusion and cell metabolism. Mutations in MFN2 cause the neurodegenerative disease Charcot-Marie-Tooth type 2A (CMT2A). The molecular basis underlying the physiological and pathological relevance of MFN2 is unclear. Here, we present crystal structures of truncated human MFN2 in different nucleotide-loading states. Unlike other dynamin superfamily members including MFN1, MFN2 forms sustained dimers even after GTP hydrolysis via the GTPase domain (G) interface, which accounts for its high membrane-tethering efficiency. The biochemical discrepancy between human MFN2 and MFN1 largely derives from a primate-only single amino acid variance. MFN2 and MFN1 can form heterodimers via the G interface in a nucleotide-dependent manner. CMT2A-related mutations, mapping to different functional zones of MFN2, lead to changes in GTP hydrolysis and homo/hetero-association ability. Our study provides fundamental insight into how mitofusins mediate mitochondrial fusion and the ways their disruptions cause disease. Mitochondria are double-membrane organelles with varying shapes influenced by metabolic conditions, developmental stage, and environmental stimuli [1] , [2] , [3] . Their highly dynamic morphology is realized through regulated and balanced fusion and fission processes [4] , [5] . Fusion is important for the health and physiological functions of mitochondria, including complementation of damaged mitochondrial DNAs and maintenance of membrane potential [5] , [6] . Outer mitochondrial membrane (OMM) fusion is catalyzed by the dynamin-like GTPase called mitofusin (MFN) [7] , [8] . Mammals have two broadly expressed and essential mitofusins, namely MFN1 and MFN2. The two mitofusins share ~80% sequence similarity, and display a certain grade of functional redundancy in mice [9] , [10] . Despite the similarities, MFN1 and MFN2 are also reported in an in vitro study to play distinct roles in mediating mitochondrial fusion via GTPase activity [11] . Compared with MFN1, MFN2 seems more versatile, and is frequently related to human diseases. MFN2 is proposed to regulate ER–mitochondria juxtaposition [12] , [13] . During the mitophagy process, MFN2 is reported to be phosphorylated by mitochondrial PTEN-induced putative kinase 1, and then recognized by Parkin for culling damaged mitochondria [14] , [15] , [16] . Functions of MFN2 have also been suggested in several other cellular processes including ER stress, axonal transport, and cell cycle progression [17] , [18] , [19] , [20] , [21] . Mutations in MFN2 , but not MFN1 , cause most cases of Charcot–Marie–Tooth type 2A (CMT2A) disease, an incurable inherited neuromuscular disorder [22] . Emerging evidence suggests that abnormal expression of MFN2 is also associated to the onset of many other human diseases including Alzheimer’s disease, Parkinson’s disease, cardiomyopathy, diabetes, and cancer [23] , [24] , [25] , [26] , [27] , [28] , [29] , [30] . However, the structural basis for the functional diversity and pathophysiological relevance of human MFN2 remains unclear. Our recent structural studies of truncated MFN1 revealed a typical dynamin-like domain organization of mitofusins, and proposed a model for mitochondrial tethering involving intermolecular (trans ) association of G domains and subsequent GTP hydrolysis-induced power stroke [31] , [32] , [33] . Although the overall architecture of MFN2 is expected to be similar as that of MFN1, the current information is still insufficient to explain the functional discrepancy of the two mitofusins. Thus, a detailed structural analysis of MFN2 is critical to pinpoint the crucial differences between the two mitofusins on the molecular level. In addition, MFN2 and MFN1 are shown to physically contact each other in cells, and this hetero-association may play an important role in mediating mitochondrial fusion and ER–mitochondria tethering [9] , [13] , [34] , but the molecular basis of their interaction has yet to be elucidated. In this study, we address these issues by presenting crystal structures of truncated human MFN2 in different stages of the GTP turnover cycle. These structures explain how MFN2 uses a primate-only single amino acid variance and a tighter G interface, as compared with human MFN1, to allow for enduring GTPase (G) domain association even after GTP hydrolysis, a feature that is unique in the dynamin superfamily and ensures efficient membrane tethering. We also found that MFN2 is able to bind MFN1 via the G interface and performs domain rearrangement in a nucleotide-dependent manner. The structures of MFN2 enable us to visualize most of the CMT2A-related mutations in a three-dimensional landscape, and explain the unexpected diverse biochemical phenotypes of these mutants and mechanisms of MFN2-related CMT2A onset. Overall, out study greatly contributes to the understanding of MFN2-mediated cellular activities and the ways its disruption cause disease. Overall structure of truncated MFN2 We generated a modified human MFN2 construct with deletions of residues 1–21 and 401–705 (MFN2 IM ). When purified from Escherichia coli , MFN2 IM was loaded with GTP or GDP, which could be removed by an optimized purification protocol (Supplementary Fig. 1a, b ). We determined crystal structures of MFN2 IM in the nucleotide-free and GDP-bound forms at 2.8 and 2.0 Å, respectively (Fig. 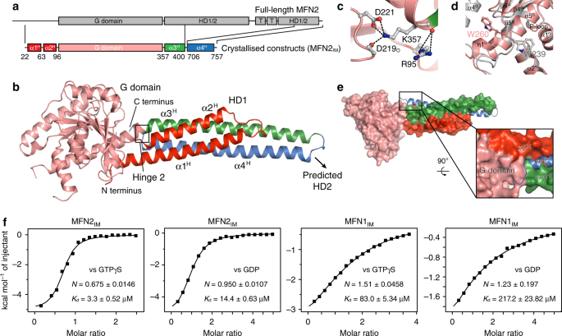Fig. 1 Overall structure of truncated MFN2IMaSchematic representation showing the organization of MFN2IMbased on full-length MFN2. G domain, GTPase domain; HD1/2, helical domain 1/2; T, transmembrane region. Elements for MFN2IMare assigned according to the structure. Borders of each element are indicated by residue numbers.bStructure of nucleotide-free MFN2IM. α-helices of HD1 are differentially colored to specify their distribution on the primary structure as ina.cDetails of hinge 2 of MFN2IMin nucleotide-free state.dStructural comparison between Trp260 in MFN2IM(pink) and Trp239 in MFN1IM(gray) in nucleotide-free states.eThe C terminus of ɑ4Hphysically contacts the G domain. Nucleotide-free MFN2IMis illustrated here.fBinding affinities (dissociation constant,Kd) to guanine nucleotides for nucleotide-free MFN2IMand MFN1IMmeasured by isothermal titration calorimetry (ITC) 1a, b , Table 1 ). MFN2 IM contains a G domain and a helical domain 1 (HD1). HD1 is connected to the G domain via the so-called hinge 2, namely Arg95 at the C-terminal end of α2 H , and Lys357 between α5 G and α3 H (Fig. 1c ). The G domain consists of a central nine-stranded β-sheet (β1 G –β6 G and β1′ G –β3′ G ) surrounded by seven ɑ-helices (ɑ1 G –ɑ5 G , ɑ1′ G , and ɑ2′ G ) and two 3 10 -helices (η1 G and η2 G ), of which β2′ G and η1 G are not observed for MFN1 IM (Supplementary Fig. 2a ). Unlike MFN1, MFN2 IM has a disordered switch I in the nucleotide-free state, and the Trp260 does not occupy the nucleotide-binding pocket (Fig. 1d ). The four-helical-bundle HD1 is stabilized by a massive hydrophobic network (Supplementary Fig. 2b ). ɑ4 H , which comprises large portion of the conventional HR2, is substantially involved in this network. The C-terminal tip of ɑ4 H physically contacts the G domain (Fig. 1e , Supplementary Fig. 2c ). With more residues preserved than in the crystallized MFN1 IM construct [32] , ɑ3 H and ɑ4 H are extended in MFN2 IM (Fig. 1b , Supplementary Fig. 2d ). A recently predicted MFN2 model proposed intramolecular interactions for Met376-Leu727, and for His380-Asp725 between ɑ3 H and ɑ4 H [35] . In our crystal structures, however, Met376 is surrounded by Phe56, Leu57, and Leu734 from the neighboring helices, and separated from Leu727. His380 and Asp725 are both on the surface, but their side chains are not close enough to form a salt bridge (Supplementary Fig. 2e ). Fig. 1 Overall structure of truncated MFN2 IM a Schematic representation showing the organization of MFN2 IM based on full-length MFN2. G domain, GTPase domain; HD1/2, helical domain 1/2; T, transmembrane region. Elements for MFN2 IM are assigned according to the structure. Borders of each element are indicated by residue numbers. b Structure of nucleotide-free MFN2 IM . α-helices of HD1 are differentially colored to specify their distribution on the primary structure as in a . c Details of hinge 2 of MFN2 IM in nucleotide-free state. d Structural comparison between Trp260 in MFN2 IM (pink) and Trp239 in MFN1 IM (gray) in nucleotide-free states. e The C terminus of ɑ4 H physically contacts the G domain. Nucleotide-free MFN2 IM is illustrated here. f Binding affinities (dissociation constant, K d ) to guanine nucleotides for nucleotide-free MFN2 IM and MFN1 IM measured by isothermal titration calorimetry (ITC) Full size image Table 1 Crystallographic data collection and refinement Full size table We tested the association of nucleotide-free MFN2 IM and MFN1 IM with different guanine nucleotides by isothermal titration calorimetry (ITC). MFN2 IM showed much higher affinity to GTPγS and GDP compared with MFN1 IM , and could efficiently bind to GMPPNP (Fig. 1f , Supplementary Fig. 2f ). The stronger nucleotide association of MFN2 IM may be partly explained by the aforementioned conformational variance to MFN1 IM : the disordered switch I and outwardly oriented Trp260 leave an empty pocket that facilitates nucleotide docking (Fig. 1d ). Thr111 in the P-loop of MFN2 has been reported to be a phosphorylation site [16] . To investigate how Thr111 phosphorylation affects the function of MFN2, we solved the crystal structure of a phosphorylation mimic MFN2 IM (T111D) (Supplementary Fig. 3a ). According to the structure, the side chain of Asp111 is not fully exposed, and its phosphorylation may require a substantial local conformational rearrangement. Phosphorylated Thr111, as reflected by the Asp111 in the crystal structure, blocks the binding groove for GTP in the P-loop, and the negative charge is also disfavored for the phosphate groups of the nucleotide (Supplementary Fig. 3b ). Subsequent ITC analysis confirmed that MFN2 IM (T111D) has no binding affinity to guanine nucleotides (Supplementary Fig. 3c ). Therefore, the putative phosphorylation at Thr111 is likely to directly inactivate MFN2 in mediating mitochondrial fusion. Intriguingly, we observed calcium ions (Ca 2+ ) associated with the HD1 of both nucleotide-free wild-type MFN2 IM and MFN2 IM (T111D), and one of them is involved in intermolecular contact (Supplementary Fig. 3d ). Addition of Ca 2+ did not alter the biochemical features of wild-type MFN2 IM or MFN2 IM (T111D) (Supplementary Fig. 3e, f ). MFN2 IM is an extremely weak GTPase Previous study showed that at low protein concentration (~0.06 μM), human MFN2 has eightfold lower GTPase activity than MFN1 in the presence of mild detergent [11] . We compared the GTP turnover rates between MFN2 IM and MFN1 IM at different protein concentrations. MFN1 IM showed stimulated GTP turnover, and the maximum k cat exceeded 7 min −1 in the presence of 150 mM KCl. In contrast, the GTP turnover of MFN2 IM remained less than 0.4 min −1 regardless of increasing protein concentrations in the same condition (Fig. 2a ). This huge difference in GTPase activity prompted us to check the GDP off-rates of MFN1 IM and MFN2 IM by fast kinetics analysis. In stopped-flow experiments, the GDP off-rate for MFN2 IM was slower than that of MFN1 IM by 13-fold (Fig. 2b ). Thus, the weak GTPase activity of MFN2 can be partly explained by the less efficient nucleotide exchange, which is also in agreement with its higher binding affinity to guanine nucleotides (Fig. 1f ) Fig. 2 MFN2 is a weak GTPase. a GTP turnover rates of MFN2 IM and MFN1 IM were measured at seven different protein concentrations. Error bars indicate s.d. ( n = 3). b GDP off-rates of MFN2 IM and MFN1 IM . A representative trace from three independent experiments is shown for each sample. c Sequence alignment of the P-loop and switch I of mitofusins from various species. Conventional motifs/residues are highlighted in green. Residues that differ between human MFN1 and MFN2 and may be responsible for GTP binding and hydrolysis are highlighted in red. hs Homo sapiens, bt Bos taurus, mm Mus musculus, ; dm Drosophila melanogaster, sc Saccharomyces cerevisiae, np Nostoc punctiforme . d GTP turnover rates of wild-type human (hs) and mouse (mm)MFN1 IM /MFN2 IM , and indicated mutants. Error bars indicate s.d. ( n = 3). e GDP off-rates of MFN2 IM (T129I) and MFN1 IM (I108T). Source data are provided as a Source Data file Full size image We then investigated the reasons for these differences between the two homologs. Human MFN1 and MFN2 bear several different residues in the P-loop and switch I, namely MFN2-Asn107/MFN1-Ser86, MFN2-Thr111/MFN1-Ser90, and MFN2-Thr129/MFN1-Ile108 (Fig. 2c ). We individually swapped corresponding residues between MFN1 IM and MFN2 IM , and applied these mutants to GTP hydrolysis assays. MFN2 IM (T129I) strongly promoted GTP turnover by ~11-fold, while MFN1 IM (I108T) showed a 12-fold decrease (Fig. 2d ). The other two swapping pairs, by contrast, did not significantly alter the GTPase activity of their wild-type counterparts (Supplementary Fig. 4a ). Interestingly, rodent MFN1 and MFN2 both have a threonine at the corresponding position in switch I (Fig. 2c , Supplementary Fig. 4b ). Mouse MFN1 IM and MFN2 IM showed weak GTPase hydrolysis similar to human MFN1 IM (I108T) and human MFN2 IM , respectively (Fig. 2d ). These results suggest that the MFN2-Thr129/MFN1-Ile108 difference in switch I is a key determinant for the incongruent GTPase activity of human mitofusins. We have previously reported that MFN1-Ile108 is involved in a hydrophobic cluster that stabilizes switch I in a nucleotide-occluding conformation [32] . The cluster is apparently disfavored by the Thr129 exchange in MFN2, which endows the observed flexibility to switch I in the nucleotide-free state (Supplementary Fig. 4c ). This idea was supported by the fact that T129I swapping in MFN2 IM slightly reduced binding affinity to GTPγS and GDP, and increased GDP off-rate, whereas MFN1 IM (I108T) led to opposite outcome (Fig. 2e , Supplementary Fig. 4d ). This moderate influence, however, seems insufficient to explain the large variance in the GTPase activity between MFN1 and MFN2. In addition, we noticed that in all ITC results of MFN2 IM , including MFN2 IM (T129I), the N values (indicating numbers of binding site) are between 0.5 and 1, whereas for MFN1 IM samples the N values are all ranged from 1 to 1.5 (Fig. 1f , Supplementary Figs. 2f, 4d ). For MFN1 IM constructs, the larger apparent N values might be derived from the conformation rearrangement of the Trp260 switch and switch I required for nucleotide loading [32] , but this does not explain the smaller N values of MFN2 IM in ITC experiments. Thus, there may be other factors that define the GTP turnover efficiency of human mitofusins, such as the dimerization of the GTPase domains. MFN2 IM remains dimerized after GTP hydrolysis Dynamin superfamily members including MFN1, are known to form functional G domain-mediated dimers in a nucleotide-dependent manner [32] , [36] , [37] , [38] . As revealed by right-angle light scattering (RALS), MFN2 IM stayed monomeric in the nucleotide-free (apo) and GDP/GTPγS/GMPPNP-loading states, and formed stable dimers in the presence of GTP or \({\mathrm{GDP}} \bullet {\mathrm{BeF}}_{3}^{-}\) (Supplementary Fig. 5a ). The MFN2 IM -GTP dimers were sustained after further incubation while the GTP was slowly hydrolyzed to GDP (Supplementary Fig. 5b ). For the MFN2 IM crystals that yielded the GDP-bound structure, the GDP was not added during purification or crystallization, but co-purified from the host E . coli cells (Supplementary Fig. 1a ). Somewhat unexpectedly, this GDP-bound MFN2 IM forms a G domain-mediated dimer across the asymmetric units of the crystal lattice (Fig. 3a and Table 1 ). RALS analysis revealed that the majority of freshly purified MFN2 IM molecules were indeed in the dimeric form (Supplementary Fig. 5c ). These observations indicate that MFN2 IM dimerizes during GTP hydrolysis, and the dimer remained associated after the reaction. In the crystal structure, two citrate ions were present between the associated G domains, and making contacts with both of them in a symmetrical manner (Supplementary Fig. 5d, e ). In solution, however, citrate did not affect GTP hydrolysis, or induce dimerization of GDP-bound MFN2 IM (Supplementary Fig. 5f, g ), suggesting that the MFN2 IM -GDP dimer in the crystal structure is not dependent on citrate. Fig. 3 Dimerization of MFN2 IM via the G domain. a The MFN2 IM dimer in GDP-bound state, with transparent surface representation. Molecule A is colored as in Fig. 1b , molecule B is in gray. GDP is shown as yellow spheres. b , Switch I configuration of MFN2 IM -GDP structure and MFN1 IM (Protein Data Bank code 5YEW) in the transition state. Switch I is colored yellow. The catalytic residues MFN2 IM (Thr130) and MFN1 IM (Thr109) are shown as ball-and-stick models. c Details of the G interface of MFN2 IM . Only one side of the G interface is shown for other involved residues except for the central dual salt bridges. d Structural comparison of MFN2 IM -GDP dimer with MFN1 IM - \({\mathrm{GDP}} \bullet {\mathrm{BeF}}_{3}^{-}\) dimer (PDB code 5YEW, left) and with MFN1 IM -GDP dimer (PDB code 5GOM, right). The structures are superimposed for one polypeptide chain (Mol A, shown in gray). The positions of the other chain (Mol B) showed a clear difference in orientation between MFN2 IM (pink) and MFN1 IM structures (light blue or green). Comparison of the G interface of MFN2 IM in the GDP-bound state ( e ) between MFN1 IM in the transition state ( f PDB code 5YEW) and in the GDP-bound state ( g PDB code 5GOM). Note the MFN2-specific Glu266-Lys307 salt bridge and the tighter trans association Full size image The area of the MFN2 IM -GDP dimeric interface (G interface) excluding citrate ions is 1065 Å 2 , which exceeds the 984 Å 2 interface of the MFN1 IM -GDP dimer of the posttransition state [32] . By comparing the catalytic sites between our MFN2 IM -GDP structure and MFN1 IM in the transition state (MFN1 IM - \({\mathrm{GDP}} \bullet {\mathrm{BeF}}_{3}^{-}\) ) [33] , we found that their switch I regions are very similar in overall conformations, as are the positions of the catalytic threonine (Fig. 3b ). When the G domains are superimposed, the HD1 of MFN2 IM takes an open orientation similar to the MFN1 IM -GDP dimer (Supplementary Fig. 6a ). On the G interface of MFN2 IM , the trans interactions include (i) the central dual salt bridges between Glu230 and Arg259; (ii) a hydrophobic cluster involving Ile126 on switch I and Trp260/Val273, and (iii) other hydrogen bonds and salt bridges (Fig. 3c ). These contacts (e.g., the hydrophobic cluster) are more consistent with those of the MFN1 IM - \({\mathrm{GDP}} \bullet {\mathrm{BeF}}_{3}^{-}\) dimer. Thus, our MFN2 IM -GDP dimer may represent a posttransition state right after GTP hydrolysis. On the other hand, the component monomers of the MFN2 IM dimer stay in different relative positions as compared with the MFN1 IM dimer (Fig. 3d ), which leads to some varied trans residue contacts in the G interface. For example, unlike in MFN1 IM in the transition state, Tyr269 of MFN2 IM only interacts with Asn161, but not with His168 (Fig. 3d and Supplementary Fig. 6b ). More importantly, Glu266 forms an MFN2-specific trans salt bridge to Lys307, whose side chain is in parallel with the guanine group of the nucleotide (Fig. 3e ). This association, together with the central salt bridge and η1 G , tightly enwraps the nucleotide. For MFN1 IM , corresponding residues are apparently relocated, resulting in a free space next to the nucleotide (Fig. 3f, g ). Tight G interface ensures high tethering efficiency to MFN2 The trans interactions were verified by single-point mutagenesis analysis. RALS analysis indicated that, except for MFN2 IM (V273D) which completely abolished dimerization in the transition state, most of these mutants only led to partial or negligible destabilization of MFN2 IM dimer (Fig. 4a , Supplementary Fig. 6c ). The resistance of the G interface to point mutations is in agreement with the stability of the MFN2 IM dimer. Analytical ultracentrifugation (AUC) assay revealed that the MFN2 IM dimer indeed has a much stronger trans association than MFN1 IM in the presence of \({\mathrm{GDP}} \bullet {\mathrm{BeF}}_{3}^{-}\) , reflected by an increased dimer fraction at an equal protein concentration (Fig. 4b ). We then performed a spectroscopic tethering assay. MFN2 IM or MFN1 IM were fused with MFN2 or MFN1 transmembrane domain (MFN2 IM -TM or MFN1 IM -TM), and reconstituted to liposomes (Supplementary Fig. 6d, e ). The tethering of the proteoliposomes caused solution turbidity, which was monitored by measuring the light absorbance at a wavelength of 405 nm. Once GTP was added, MFN2 IM -TM tethered liposomes in a significantly higher efficiency as compared with MFN1 IM -TM (Fig. 4c ). Fig. 4 Characterization of MFN2 IM dimeric interface. a Dimerization property of the G interface mutants in the presence of \({\mathrm{GDP}} \bullet {\mathrm{BeF}}_{3}^{-}\) was assayed by analytical gel filtration coupled to RALS. Calculated molecular masses at the absorption peaks of 280 nm are plotted in red. mAU milli-absorption units. b AUC results of MFN2 IM and MFN1 IM (theoretical molecular mass 52.6 and 50.9 kDa, respectively) in the presence of \({\mathrm{GDP}} \bullet {\mathrm{BeF}}_{3}^{-}\) . The estimated molecular masses determined by sedimentation velocity are given in kilodaltons (kDa) above the peaks. c Liposome tethering assay for wild-type MFN2 IM -TM/MFN1 IM -TM and mutants. A representative plot from three independent experiments is shown. d Dimerization via the G interface slows down the nucleotide exchange of MFN2 IM and MFN1 IM . The initial part of each fluorescence trace was magnified. e Effect of MFN2 IM (T129I) and MFN1 IM (I108T) on the nucleotide exchange efficiency in the dimeric state. The initial part of each fluorescence trace was magnified and fitted to exponential function as shown in a white curve. f Surroundings of MFN2-Thr129 and MFN1-Ile108 in the dimerization form. g Model for comparison between MFN2 and MFN1 in G domain dimerization. Note the tighter G interface of MFN2 and its sustained dimerization in the GDP-bound state. Pi denotes phosphate group. h Mitochondrial elongation assay with quantification for wild-type MFN2 and G interface mutants. Representative images are shown. Mfn 1/2-null MEFs were transduced with retrovirus expressing 16× Myc-tagged WT Mfn2 or G interface mutants. Actin was used as a loading control. A lysate from WT MEFs is shown for comparison. For each construct, 100 cells were scored in biological triplicate. Error bars indicate s.e.m. Scale bars, 10 μm. Source data are provided as a Source Data file Full size image To examine how G domain dimerization affects GTP turnover rate, we designed a nucleotide exchange assay by instantaneously mixing preincubated MFN1/2 IM -GDP (monomeric) or MFN1/2 IM - \({\mathrm{GDP}} \bullet {\mathrm{BeF}}_{3}^{-}\) (dimeric) with fluorescently-labeled GTP (mant-GTP) using stopped-flow. The initial slope of the fluorescent increase indicates the efficiency of mant-GTP reload. Although MFN2 IM bound more mant-GTP over time due to a higher affinity to GTP as compared with MFN1 IM , the mant-GTP reload to MFN2 IM was much slower. G domain dimerization greatly reduced the mant-GTP reload rate of both MFN2 IM and MFN1 IM (Fig. 4d ). MFN2 IM (T129I) and MFNI IM (I108T) showed promoted and reduced mant-GTP reload rates compared with wild-type proteins in \({\mathrm{GDP}} \bullet {\mathrm{BeF}}_{3}^{-}\) condition, respectively (Fig. 4e ), suggesting that the Thr/Ile difference also plays an important role in G domain dimerization. In consistent with this, swapping MFN1-Ile108/MFN2-Thr129 elevated tethering activity for MFN1 IM and drastically reduced it for MFN2 IM (Fig. 4c ). A structural explanation is that, compared with MFN1-Ile108, MFN2-Thr129 is more favored in the polar G interface for maintaining dimerization (Fig. 4f ). Whether interrupting dimerization or not, the G interface mutants of MFN2 IM had comparable GTP turnover with wild type (Supplementary Fig. 6f ). Altogether, the tight trans interaction within MFN2 dimer is likely to confine the conformational dynamics of switch I and prevent the reload of GTP, which ultimately accounts for the low GTP turnover rate (Fig. 4g ). On the other hand, living cells seem quite sensitive to mutations in the G interface, as mutants I126D, N161A, and K307A were highly defective in mitochondrial elongation assays, although some residual activity remained (Fig. 4h ). MFN2 interacts with MFN1 via the G interface Surface conservation analysis using 12 mitofusin sequences from zebra fish to human revealed that the G interface is a highly conserved area in mitofusins (Fig. 5a ). Given the fact that MFN1 and MFN2 share many key residues for G domain dimerization, we postulated that the G interface is involved in the formation of mitofusin hetero-complexes. To explore this idea, we performed pull-down assays in different nucleotide-loading conditions. MFN2 IM substantially co-eluted with glutathione S-transferase (GST)-tagged MFN1 IM in the presence of GTP or \({\mathrm{GDP}} \bullet {\mathrm{BeF}}_{3}^{-}\) . GDP also led to weak association between the two proteins, but this hetero-association was not observed in apo or GTPγS-bound conditions (Fig. 5b ). The G interface mutants MFN2 IM (E230A) and MFN2 IM (R259A) failed to interact with their MFN1 IM counterparts (Fig. 5c ). When maltose-binding protein (MBP)-fused MFN1 IM and His 6 -tagged MFN2 IM were mixed together with \({\mathrm{GDP}} \bullet {\mathrm{BeF}}_{3}^{-}\) , the MFN1 IM –MFN2 IM heterodimer was efficiently formed and could be stably purified (Fig. 5d, e ). The hydrolysis-deficient MFN2 IM (T130A) was able to stimulate the GTP turnover of MFN1 IM in a similar manner to MFN1 IM self-stimulation [32] , and the introduction of two G interface mutations significantly weakened this effect (Fig. 5f ). Liposomes that carry MFN1 IM fused with a transmembrane domain of Sac1 (MFN1 IM -TM Sac1 ) were able to tether MFN2 IM -TM Sac1 -associated liposomes in the presence of GTP or \({\mathrm{GDP}} \bullet {\mathrm{BeF}}_{3}^{-}\) , and the tethering was disrupted by the G interface mutants (Fig. 5g ). Fig. 5 MFN2 interacts with MFN1 via G domain. a Surface conservation analysis reveals that the G interface is a highly conserved area in mitofusins. b Pull-down assays showing the interaction between MFN2 IM and GST-tagged MFN1 IM in different nucleotide-loading conditions. c Pull-down assays showing that the interaction between MFN2 IM and MFN1 IM is dependent on the G interface. d Native PAGE result showing the association between MFN2 IM and MBP-fused MFN1 IM . e SDS-PAGE showing the purified MFN2 IM /MBP-MFN1 IM hetero-complex. f MFN2 IM stimulates GTP turnover of MFN1 IM . Overall, 0.25 μM MFN1 IM and 2.5 μM MFN1 IM MFN2 IM mutants were used. g Liposome tethering assay for wild-type MFN2 IM /MFN1 IM and G interface mutants. Representative images from five independent experiments are shown. Scale bar, 50 μm. h FRET experiment showing the G domain dimerization-dependent conformational change of MFN2 IM in different nucleotide-loading conditions. The time point for the addition of corresponding nucleotides is indicated by an arrow for each panel. nt denotes nucleotide. i FRET experiment showing the conformational change of MFN2 IM and MFN1 IM upon association via the G domains in GTP- and \({\mathrm{GDP}} \bullet {\mathrm{BeF}}_{3}^{-}\) loading conditions. j A model for the trans association between MFN2 IM and MFN1 IM . Source data are provided as a Source Data file Full size image MFN1 IM was shown to have conformational dynamics coupled to the GTP turnover cycle [33] . In the transition state, the MFN1 IM dimer bends via the hinge 2, and the two HD1s move close to each other. This domain rearrangement can be monitored by FRET changes between labeled residues at appropriate positions. To understand whether MFN2 IM also has this feature, we introduced Cy3/Cy5 labels to MFN2 IM at the distal end of HD1 (Supplementary Fig. 7a–d ), and traced the ensemble FRET in different nucleotide-loading states. Addition of GTP, \({\mathrm{GDP}} \bullet {\mathrm{BeF}}_{3}^{-}\) , or GDP induced immediate FRET increase, whereas G interface mutants had no FRET change in all conditions (Fig. 5h ). Similarly, mixture of differentially labeled MFN1 IM and MFN2 IM also exhibited FRET increase when GTP or \({\mathrm{GDP}} \bullet {\mathrm{BeF}}_{3}^{-}\) was supplied, and this FRET increase was apparently dependent on the G interface (Fig. 5i ). These results confirmed that MFN2 confers domain rearrangement, and can associate with MFN1 via the G interface in a nucleotide-dependent manner (Fig. 5j ). Structural and biochemical investigations of CMT2A mutations Mutations in the Mfn2 gene are main cause of CMT2A. Most of these mutations result in single amino substitutions that are mainly distributed in the G domain and HD1. Although some CMT2A-related MFN2 mutations have been studied based on MFN1 structures [31] , [33] , more accurate conclusions require comprehensive analysis using a bona fide human MFN2 structure as the two mitofusins display substantial difference in the organization of G interface and GTPase activity. We plotted reported CMT2A mutations on the MFN2 IM structural model. The majority of them are on the surface of the protein (Fig. 6a ). For example, the frequently mutated residues Arg104, Thr105, Gln276, and Arg280 are distributed around the G interface (Supplementary Fig. 8a ). Arg94 is neighboring the hinge 2 linking G domain and HD1 (Supplementary Fig. 8b ). Arg364 and Trp740 are on the surface of HD1 (Supplementary Fig. 8c ). These surface-exposed disease-related residues are not involved in the intramolecular interactions, except that Arg104 forms a salt bridge with Asp204 in the GDP-bound state (Supplementary Fig. 8d ). Overall, most of these mutations are not likely to severely disrupt folding of MFN2, as was corroborated by circular dichroism (CD) analysis (Supplementary Fig. 8e ). Fig. 6 Characterization of CMT2A-related mutants. a Overview of the CMT2A-mutation sites on MFN2. The CMT2A-related single-point mutation sites are specified as yellow spheres on MFN2 IM structure colored as in Fig. 1b . b GTP turnover rates of selected CMT2A-related MFN2 IM mutants in comparison with wild-type MFN2 IM . Locations of these mutants are color-specified. c CMT2A-mutation sites on the putative G domain-HD1 contact of MFN2 in the transition state. The structural model of rearranged MFN2 IM is generated base on the MFN1 IM - \({\mathrm{GDP}} \bullet {\mathrm{BeF}}_{3}^{-}\) structure (PDB code 5YEW). CMT2A-related residues and their potential interaction partners are presented as ball-and-stick models. d Functional zones of MFN2 and the involved CMT2A-mutation sites. e Dimerization property of CMT2A-mutants on the putative G domain-HD1 interface in the presence of \({\mathrm{GDP}} \bullet {\mathrm{BeF}}_{3}^{-}\) . Source data are provided as a Source Data file Full size image To explore the biochemical influence of these mutations, we tested 20 MFN2 IM constructs, each with a CMT2A-related mutation distributed in various regions of MFN2. Interestingly, over half of the mutants showed elevated GTPase activity compared with wild type, suggesting that slow GTP turnover is a crucial attribute for MFN2’s physiological function. Of these mutants, T105M and N131S are either on the P-loop or Switch I, and thus their direct influence on GTP turnover is intuitive. In contrast, L248V and P251L on the G domain, R94W and R94Q on the hinge 2, as well as R364P and R364W on HD1 are all distant from the catalytic site but strongly promoted GTP turnover (Fig. 6b ). By referring to the \({\mathrm{GDP}} \bullet {\mathrm{BeF}}_{3}^{-}\) -bound structure of MFN1 IM [33] , we noted that Leu248, Pro251, and Arg364 are likely involved in the putative interface between the G domain and the reoriented HD1 (Fig. 6c, d ). For example, Arg343 in MFN1, which is equivalent to MFN2-Arg364, forms a hydrogen bond with Asn224. Mutagenesis of these residues would disrupt this interface, thereby intervening the relative movement of G domain and HD1. R94W and R94Q are also expected to disturb the conformational dynamics of MFN2. These six mutants did not significantly perturb dimerization via the G interface (Fig. 6e ), while some of their counterparts on MFN1 do [33] . This highlights a direct mechanistic coupling between the GTPase activity and domain rearrangement for MFN2 regardless of nucleotide-dependent dimerization, and may be relevant to a recent observation that a R364W-like mutation causes excessive mitochondrial fusion in a Drosophila model [39] . While some CMT2A-related mutations occurring at the G interface (R104W, T105M, G127V) prevent the dimer formation in the transition state of GTP hydrolysis, other mutants could still dimerize (Supplementary Fig. 8f ). To further test whether they are able to associate with wild-type mitofusins via G domains, we individually mixed the mutants with either MBP-fused MFN2 IM or MFN1 IM in the presence of GDP•BeF 3 − . Native PAGE analysis indicated that except those on the G interface, the majority of the CMT2A-related mutants efficiently heterodimerized with wild-type MFN2 IM or MFN1 IM (Fig. 7a ). The R94W mutant, as an example, even formed no homodimers but only heterodimers with wild-type MFN2 or MFN1, which coincides with a previous co-immunoprecipitation study in human U2OS cells [40] . This implicates that corresponding mutations may have a dominant negative effect on the occurrence of CMT2A. The structural and biochemical information of available CMT2A-related mutations is summarized in Supplementary Table 1 . Fig. 7 Interaction between CMT2A-related mutants and wild-type MFN1/2 IM . a G domain-mediated association of CMT2A-related MFN2 IM mutants with MBP-fused MFN2 IM (upper) or MBP-MFN1 IM (lower) tested by native PAGE. b Schematic drawing showing the two causes of CMT2A onset that may be derived from different MFN2 mutations. Source data are provided as a Source Data file Full size image MFN2 and its homologs play pivotal roles in mitochondrial homeostasis and cell metabolism from yeast to human. Our study reveals the structural and biochemical features of this key molecule that underlie its divergent functions. MFN2 possesses most of the traits of the dynamin superfamily such as domain organization and G domain-mediated dimerization. However, unlike almost all other members (including human MFN1) with dimerization-stimulated GTPase activity that entails frequent attaching–detaching cycles of the G domains coupled with multiple rounds of GTP hydrolysis, MFN2 has a hydrolyze-but-not-dissociate feature. Keeping basal (low) GTP turnover seems crucial for the cellular function of MFN2, as many GTPase activity-promoting mutants are associated with CMT2A onset. Of these mutants, T105M and P251L have been previously shown to lack fusogenic activity [41] . The more stable G domain dimerization and potent tethering activity, as compared with human MFN1 in our experiment, imply that MFN2 may act as a GTP-regulated molecular sticker for mitochondria. GTP-loaded MFN2 molecules may be able to establish enduring trans anchoring of juxtaposing mitochondria throughout hydrolysis cycle. Although MFN2 has been previously reported to bear weaker tethering activity than MFN1 [11] , the isolated MFN2 used in the tethering experiment may already have been loaded with host GDP. Thus, it is tempting to speculate that MFN2 molecules serve as initial mitochondrial anchors in the beginning of the fusion process. The free and vigorous relative movement between HD1 and HD2 via hinge 1, as found also in dynamin-like MxA and bacterial DLPs [42] , [43] , [44] , may draw the tethered mitochondrial segments together. This proposed mechanism is economic in GTP consumption, thereby ensuring that mitochondrial tethering can happen at low local MFN2 or GTP concentrations. Given the tight G interface of MFN2, it is possible that external partners, such as the Smad2-RIN1 complex that are reported to promote GTP turnover of MFN2 [45] , help with G domain dissociation after GTP hydrolysis. Other cellular factors may also participate in the regulation of MFN2: the potential of binding Ca 2+ and citrate found in the crystal structure implies a possibility of physiological relevance between MFN2 and these molecules. It has been recently reported that Ca 2+ affects mitochondrial fusion by inhibiting MFN1 assembly [46] , and citrate is known to be transported to cytoplasm from Krebs cycle and modulate acetyl-CoA carboxylase for fatty acid metabolism [47] . Can they somehow influence OMM fusion through direct interaction with MFN2 in living cells? It may be worthwhile to explore these ideas. A following question is whether the tethering efficiency of MFN2 translates to high fusogenic activity. On one hand, tight dimerization and resulting low GTP turnover rate of MFN2 may not favor mitochondrial fusion, as the fusion event requires continuous GTP hydrolysis cycles. Firmly trans -associated MFN2 molecules stacking between two segments of mitochondrial outer membrane may even prevent their contact. On the other hand, if these trans -associated MFN2 molecules are organized in so-called docking ring complexes as reported earlier in an in vitro assay for yeast Fzo1 [48] , mitochondrial fusion may be promoted. We used internally truncated MFN1/2 variants in liposome tethering assays, and they lack the HD2 region which is indispensible for fusion. Although previous studies showed that MFN1/2 (or Fzo1) are able to fuse mitochondria in vitro by using mitochondria isolated from mouse embryonic fibroblasts (MEFs) [49] or yeast [48] , one cannot exclude the possibility that these mitochondria carry other adapters (specific lipids or proteins) that are essential for fusion. To understand whether MFN2 (or MFN1) on its own can efficiently catalyze mitochondrial outer membrane fusion, an in vitro fusion assay using full-length mitofusin and clean mitochondria (or liposomes) will be needed. The difference between human MFN1 and MFN2 in GTP turnover efficiency largely derives from the Ile108/Thr129 variance, which can lead to difference in the flexibility of switch I and also in the stability of G interface. By careful sequence screening, we found that this single amino acid variance of MFN1/2 only exists in primates (Supplementary Fig. 4b ). In this context, the particularly high GTPase activity of human MFN1, as compared with other mitofusins, suggests that primates may have special needs for mitochondrial fusion. In line with these ideas, MFN1 in nonprimate mammals is likely to share more functional redundancy with MFN2 as they do not display the Ile/Thr variance in switch I. As currently there is no MFN1 knockout data for primates, the question why MFN1 mutations are not found to be clearly related with human diseases, say CMT2A, may have two distinct answers: (i) primate MFN2 is unable to compensate for defective MFN1, and detrimental mutations in MFN1 cause death in early embryonic development; (ii) primate MFN2 can efficiently substitute defective MFN1 but not vice versa, therefore only defects in MFN2 lead to disease. Given this functional complexity, the physiological role of MFN1 in humans needs to be dissected in more detail, and proper animal models are required. The heterodimerization between human MFN2 and MFN1 found in our study is likely to occur in trans and compete with homotypic MFN1/MFN2 associations during mitochondrial fusion as the two types of interactions are both mediated by the G interface. According to the native PAGE results, the tendency of MFN1–MFN2 heterodimerization in vitro is even stronger than that of homodimerization (Figs. 5d , 7a ). If this is true also for mouse mitofusins, it may partly explain the previous observation that heterotypic MFN1/MFN2 trans complexes show greater fusogenic efficacy in MEFs as compared with homotypic MFN1 or MFN2 complexes [49] . It is important to investigate the particular physiological role of this heterodimerization in OMM fusion and ER–mitochondria tethering in vivo in the future, and our results contribute to the development of more efficacious methodologies for this purpose. Based on our CD spectroscopy experiments, the majority of reported CMT2A-related missense mutations do not seem highly detrimental to protein folding. Some of these mutants may even preserve a certain level of functionality in OMM fusion. These mutations can be mapped to at least four functional zones of the molecule, including (I) the nucleotide-binding site (the P-loop, Switch I/II and G4 motif), (II) G interface, (III) hinge 2, and (IV) G domain-HD1 interface (Fig. 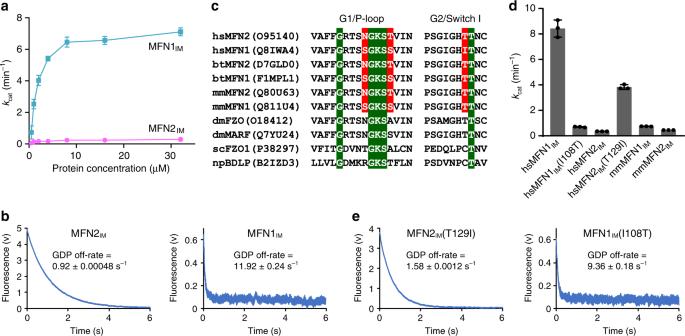Fig. 2 MFN2 is a weak GTPase.aGTP turnover rates of MFN2IMand MFN1IMwere measured at seven different protein concentrations. Error bars indicate s.d. (n= 3).bGDP off-rates of MFN2IMand MFN1IM. A representative trace from three independent experiments is shown for each sample.cSequence alignment of the P-loop and switch I of mitofusins from various species. Conventional motifs/residues are highlighted in green. Residues that differ between human MFN1 and MFN2 and may be responsible for GTP binding and hydrolysis are highlighted in red. hsHomo sapiens,btBos taurus,mmMus musculus,; dmDrosophila melanogaster,scSaccharomyces cerevisiae,npNostoc punctiforme.dGTP turnover rates of wild-type human (hs) and mouse (mm)MFN1IM/MFN2IM, and indicated mutants. Error bars indicate s.d. (n= 3).eGDP off-rates of MFN2IM(T129I) and MFN1IM(I108T). Source data are provided as a Source Data file 6d , Supplementary Table 2 ). The consequence of these mutations in these zones can therefore be predicted from the biochemical feature of MFN2. For example, R104W of the nucleotide-binding site, R94W of hinge 2 and R364P of the G domain-HD1 interface all cause severe CMT2A phenotype, whereas the dominant L745P and Q276R mutations, which are beyond the above four functional zones, only lead to mild or moderate disease conditions [50] . It is also possible that, mutations of residues beyond these zones but involved in critical interaction with other partners of MFN2, also results in severe CMT2A phenotype. Different mechanisms for MFN2-related CMT2A occurrence are also expected on the intermolecular level. The dimerization-deficient T105M mutant is highly defective in promoting mitochondrial fusion [41] , but it is less likely to affect the functionality of wild-type MFN1 and MFN2, at least in terms of G domain association. Consequently, the development of the CMT2A phenotype in T105M patients are likely due to reduced cellular level of normal MFN2. This mechanism possibly also applies to MFN2 mutations that lead to unfolded or truncated proteins. On the other hand, those mutants that are still able to dimerize and retain residual fusogenic activity, as compared with MFN2(T105M), tend to have a dominant negative effect through hijacking normal MFN1 and allelic MFN2, which eventually results in a pervasively weakened MFN2 and MFN1 activity (Fig. 7b ). In this case, the level of retained fusogenic activity of the mutant is a key determinant for the onset of the disease. Altogether, this information will be valuable for the diagnosis and prognosis of CMT2A cases, and for the development of personalized treatments targeting particular MFN2 mutations. Protein expression and purification The engineered MFN2 construct (MFN2 IM ) was cloned into a modified pET-28 vector. Details of this construct are illustrated in Fig. 1a . All mutants were generated by site-directed mutagenesis. Primer sequences for amplification and cloning here are provided in Supplementary Table 2 (primers 1–4). Recombinant MFN2 IM proteins containing an N-terminal His 6 -tag followed by a cleavage site for PreScission protease (PSP) were expressed in E. coli Rosetta (DE3) cells (Invitrogen). Transformed bacteria were cultured at 37 °C before induced with 0.1 mM isopropyl-1-thio-β-d-galactopyranoside (IPTG) at an OD 600 nm of 0.6, and grown for 20–24 h at 17–18 °C in Terrific Broth medium. Initially, human MFN2 IM was purified following our previous protocol for MFN1 IM [32] , which was used for obtaining GDP-bound MFN2 IM crystals. To remove host-derived nucleotides bound to MFN2 IM , cells were lysed in 50 mM HEPES, pH 7.5, 1 M NaCl, 30 mM imidazole, 2.5 mM β-mercaptoethanol (β-ME), 1 μM DNase I, and 1 mM phenylmethanesulfonylfluoride (PMSF) using a cell disruptor (JNBIO) and subjected to centrifugation at 40,000 g for 50 min. The supernatant was filtered and applied to an Ni-NTA (first Ni-NTA) column (GE Healthcare) equilibrated with buffer A containing 20 mM HEPES, pH 7.5, 1 M NaCl, 30 mM imidazole, and 2.5 mM β-ME. After washed with buffer A, protein was eluted with 20 mM HEPES, pH 7.5, 1 M NaCl, 300 mM imidazole, and 2.5 mM β-ME. Eluted proteins were incubated with 20 μg glutathione S-transferase (GST)-fused PSP to remove the His 6 -tag and dialyzed overnight against buffer B containing 20 mM HEPES, pH 7.5, 800 mM NaCl, 2.5 mM β-ME. After dialysis, PSP was removed by a GST column. The protein was reapplied to a second Ni-NTA column equilibrated with buffer B and eluted with buffer A, and further purified by gel filtration chromatography (Superdex 200 16/60 column, GE Healthcare) in buffer C containing 20 mM HEPES, pH 7.5, 150 mM KCl, 5 mM MgCl 2 , and 1 mM dithiothreitol (DTT). For nucleotide-free MFN2 IM used in crystallization experiments, KCl was substituted by NaCl in buffer C during gel filtration. His 6 -tagged MFN1 IM and mutants were purified as previously described [32] . Cells expressing MFN1 IM or mutants were lysed in 50 mM HEPES, pH 7.5, 400 mM NaCl, 5 mM MgCl 2 , 30 mM imidazole, 1 μM DNase I, 1 mM PMSF, and 2.5 mM β-ME and subjected to centrifugation at 40,000 g for 1 h. The supernatant was filtered and applied to a Ni-NTA (first Ni-NTA) column (GE Healthcare) equilibrated with binding buffer D containing 20 mM HEPES, pH 7.5, 400 mM NaCl, 5 mM MgCl 2 , 30 mM imidazole, and 2.5 mM β-ME. After washed with binding buffer D, proteins were eluted with elution buffer containing 20 mM HEPES, pH 7.5, 400 mM NaCl, 5 mM MgCl 2 , 300 mM imidazole, and 2.5 mM β-ME. Eluted proteins were incubated with 20 μg GST-fused PSP to remove the His 6 -tag and dialyzed overnight against binding buffer E containing 20 mM HEPES, pH 7.5, 400 mM NaCl, 5 mM MgCl 2 , and 2.5 mM β-ME. After dialysis, PSP was removed using a GST column. The protein was reapplied to a second Ni-NTA column equilibrated with binding buffer E. Binding buffer D was used to elute the proteins which were subsequently loaded onto a Superdex 200 16/60 column (GE Healthcare) equilibrated with gel filtration buffer C. Cell lysis and protein purification were both performed at 4 °C. E. coli cells expressing GST- and MBP-fused MFN1 IM (recombinant in pGEX-6p-1 vector or a modified MBP vector, a gift from Professor Tengchuan Jin), as well as corresponding mutants, were cultured and lysed in similar protocols as His 6 -tagged MFN1 IM construct, but the lysis buffer contains no imidazole. In the affinity chromatography experiments, elution buffer contains either 15 mM reduced glutathione (GSH) for GST-fused MFN1 IM , or 10 mM maltose for MBP-fused MFN1 IM . The protein was purified by gel filtration chromatography in buffer C. All cell lysis and protein purification performances were carried out at 4 °C. Primer sequences for amplification and cloning here are provided in Supplementary Table 2 (primers 27 and 32 for pGEX-6p-1 vector; primers 5–8 for MBP vector). For transmembrane domain (TM)-fused MFN1 IM or MFN2 IM used in spectroscopic tethering assay. The original residues 365–694 of MFN1 were replaced with the TM of codon-optimized MFN1 (residues 596–628) flanked by amino acid sequences SGSGSGGS (N-terminal) and GSGS (C-terminal) using overlap PCR. The original residues 401–705 of MFN2 were replaced with the TM of MFN2 (residues 615–647) flanked by SAASA (N-terminal) and ASAA (C-terminal). The fragments were individually cloned into the pGEX-6p-3 vector. Primer sequences for amplification and cloning here are provided in Supplementary Table 2 (primers 9–20). All point mutations were generated by site-directed mutagenesis. MFN1 IM -TM, MFN2 IM -TM and corresponding mutants were expressed and purified as previously described [33] . Plasmids expressing MFN1 IM -TM or MFN2 IM -TM were transformed into E. coli BL21 (DE3). Cells were grown to an OD 600 nm of 0.8, induced with 0.3 mM IPTG for 24 h at 16 °C, and harvested by centrifugation. The pellets were resuspended in buffer F containing 25 mM HEPES, pH 7.4, 150 mM NaCl, 10% glycerol, 1 mM EDTA, and 2 mM β-ME. Membranes were then pelleted by centrifugation at 110,000 g for 1 h, and dissolved by 1% Fos-choline-12 (Anatrace) in buffer F, and insoluble components were cleared by centrifugation. The recombinant protein was isolated by glutathione Sepharose (GE Healthcare), washed twice with buffer F containing 0.1% Triton X-100 (Anatrace), and the GST-tag was cleaved before reconstitution. For constructs used in visual tethering assay, the TM of Sac1 (residues 523–580) was inserted between α3 H and α4 H of MFN1 IM (MFN1 IM -TM Sac1 ) or MFN2 IM (MFN2 IM -TM Sac1 ) by overlapping PCR, and the fragments were individually cloned into pGEX-6p-1 vector. Primer sequences for amplification and cloning here are provided in Supplementary Table 2 (primers 21–32). MFN1 IM -TM Sac1 , MFN2 IM -TM Sac1 and corresponding mutants were expressed and purified as previously described [51] . Proteins were expressed in E. coli Rosetta (DE3) cells for 16 h at 17–18 °C. Collected cells expressing MFN1/2 IM -TM Sac1 or its mutants were lysed in 50 mM HEPES, pH 7.5, 150 mM NaCl, 30 mM imidazole, 10% glycerol, 2% Triton X-100, 1 µM DNase I, 1 mM PMSF, and 2.5 mM β-ME and centrifugated at 40,000 g for 30 min. After incubation at 4 °C for 1 h, the supernatant was subjected to further centrifugation at 40,000 g before filtered and applied to a GST column (GE healthcare) which is equilibrated with binding buffer G containing 50 mM HEPES, pH 7.5, 150 mM NaCl, 30 mM imidazole, 10% glycerol, 0.1% Triton X-100, and 2.5 mM β-ME. Target proteins were eluted with buffer G supplied with 15 mM GSH. Target proteins with GST-tags removed were reapplied to a GST column after dialysis using buffer G. Eluted target proteins were loaded onto a Superdex 200 16/60 column equilibrated with 20 mM HEPES, pH 7.5, 150 mM NaCl, 5% glycerol, 0.1% Triton X-100 and 1 mM DTT and collected. For MFN2 IM -TM Sac1 or its mutants, 1 M NaCl instead of 150 mM NaCl was used in buffer G. Protein crystallization MFN2 IM constructs were crystallized via hanging drop vapor diffusion by mixing equal volumes of protein (~20 mg ml −1 ) and reservoir solution. Crystals of nucleotide-free MFN2 IM grew from 0.19 M calcium chloride, 95 mM HEPES, pH 7.5, 26.6% PEG400, 5% glycerol at 4 °C. MFN2 IM (T111D) was crystallized in 0.16 M calcium acetate, 0.08 M sodium cacodylate pH 6.5, 14.4% PEG 8000, 20% glycerol at 18 °C. Crystals of GDP-bound MFN2 IM were grown from 0.2 M lithium citrate tribasic tetrahydrate, and 35% glycerol ethoxylate at 18 °C using MFN2 IM purified with previous protocol for MFN1 IM [32] . Structure determination X-ray diffraction datasets were collected at beamlines BL17U1 and BL19U1 of Shanghai Radiation Facility (SSRF) [52] and processed with the XDS suite [53] . Structures of MFN2 IM were solved by molecular replacement using MOLREP [54] with truncated MFN1 IM as the search model. Models were built with COOT [55] and refined with Refmac [56] and Phenix [57] . Structural validation was carried out using MolProbity [58] . Structural illustrations were prepared using the PyMOL Molecular Graphic Systems (version 0.99, Schrödinger LLC; http://www.pymol.org/ ). The Ramachandran statistics determined by PROCHECK [59] are as follows: 97.7% in favored region, 2.3% allowed, 0 outlier for apo MFN2 IM ; 98.3% favored, 1.5% allowed, 0.2% outlier for MFN2 IM (T111D) and 98.6% favored, 1.4% allowed, 0 outlier for GDP-bound MFN2 IM . Nucleotide-binding assay The equilibrium dissociation constants for nucleotide-free MFN2 IM , MFN1 IM and indicated mutants to guanine nucleotides were determined by ITC at 25 °C using a MicroCal ITC200 (Malvern) in the buffer containing 20 mM HEPES, pH 7.5, 150 mM KCl, 5 mM MgCl 2 . A total of 1–2 mM nucleotides were used to titrate 80 μM protein. Resulting heat changes upon each injection was integrated and the values were fitted to a standard single-site binding model using Origin7. GTP hydrolysis assay GTP hydrolysis assays were performed at 37 °C as previously described [32] in buffer containing 20 mM HEPES, pH 7.5, 150 mM KCl, 5 mM MgCl 2 , and 1 mM DTT. Reactions were initiated by the addition of protein to the final reaction solution. At different time points, reaction aliquots were 20-fold diluted in buffer C and quickly transferred into liquid nitrogen. Nucleotides in the samples were separated via a reversed-phase Hypersil ODS-2 C18 column (250 × 4.6 mm, Thermo), with 10 mM tetrabutylammonium bromide, 100 mM potassium phosphate, pH 6.5, and 7.5% acetonitrile as running buffer, where denatured proteins were blocked by a C18 guard column (Thermo). Nucleotides were detected by absorption at 254 nm and quantified by integration of the corresponding peaks. The GTP hydrolysis rates derived from a linear fit to the initial phase of the reaction (<40% GTP hydrolyzed) were plotted against the protein concentrations. For measuring stimulated GTP turnover of MFN2 IM and MFN1 IM , proteins at concentrations of 0.5, 1, 2, 4, 8, 16, and 32 μM were individually mixed with 1–2 mM GTP. For measuring stimulated GTP turnover of MFN1 IM by hydrolysis-deficient MFN1 IM or MFN2 IM constructs, 0.25 μM MFN1 IM and 1 mM GTP were mixed with 2.5 μM MFN2 IM (T130A) or MFN2 IM (T130A/E230A/R259A). For other experiments, 32 μM protein and 2 mM GTP were used. Fast kinetics assay To determine the GDP off-rate, 10 μM protein was preincubated with 2 μM N-methyl-3′-O-anthranoyl (mant-)GDP (Jena Bioscience) for 2 h before rapidly mixed with 1 mM unlabeled GDP in a buffer containing 20 mM HEPES, pH 7.5, 150 mM KCl, 5 mM MgCl 2 and 1 mM DTT, and the fluorescence signal (excitation wavelength 355 ± 4 nm) was instantaneously recorded using a Chirascan spectrometer equipped with an SX20 Stopped-Flow accessory (Applied Photophysics). Three injections were individually and consecutively carried out, and the readouts were averaged to yield a time-dependent fluorescence change diagram. The GDP off-rates were derived from fitting the fluorescence traces with single exponential function. For mant-GTP exchange assay, 5 μM proteins were preincubated with 50 μM GDP or 50 μM GDP•BeF 3 ¯ (50 μM GDP, 50 μM BeSO 4 , and 500 μM NaF) at room temperature for 2 h before rapidly mixed with 2 μM mant-GTP in a buffer containing 20 mM HEPES, pH 7.5, 150 mM KCl, 5 mM MgCl 2 , and 1 mM DTT. RALS A coupled RALS-refractive index detector (Malvern) was connected in line to an analytical gel filtration column Superdex 200 10/300 to determine absolute molecular masses of the applied protein samples. 50 μM purified protein was incubated with or without 500 μM corresponding ligand for 2 h at room temperature before applied to the column equilibrated with 20 mM HEPES, pH 7.5, 150 mM KCl, 5 mM MgCl 2 , and 1 mM DTT. Data were analyzed with the OMNISEC software. All experiments were repeated at least twice and the data showed satisfying consistency. Mitochondrial elongation assay To examine the effect of point mutations, MFN2–Myc variants were expressed in Mfn1 / 2 -null MEFs [10] from the pQCXIP retroviral vector. The cell line is free of mycoplasma and has been authenticated by genotyping with PCR to confirm deletion of the Mfn1 and Mfn2 genes. Point mutants in mouse Mfn2 were constructed by overlapping PCR with primers encoding the point mutation. For I126D, the 5′ region of the Mfn2 cDNA was amplified with primers 33 and 34, and subcloned as a NotI/MfeI fragment. For N161A, two overlapping Mfn2 fragments were amplified with primers 35–38 (N161A). The two fragments were combined, reamplified with primers 35 and 38, and subcloned as an MfeI/PsiI fragment. The same strategy was used to subclone K307A, except that primers 39 and 40 were used instead of primers 36 and 37. All primers used here are provided in Supplementary Table 2 . All mutations were confirmed by DNA sequencing. The types and positions of the residues mutated in this study are all consistent between human and mouse mitofusins. Retroviral supernatants were produced from 293T cells transfected with the retroviral vector and the packaging plasmid pCLEco. Mfn 1/2-null MEFs stably expressing mito-DsRed were maintained in Dulbecco’s Modified Eagle’s Medium supplemented with 10% fetal bovine serum and penicillin/streptomycin at 37 °C and 5% CO 2 . After retroviral transduction of Mfn 1/2-null MEFs, puromycin selection was applied for 2 days. Cells were plated onto eight-well chambered slides for analysis. Western blot analysis with the 9E10 antibody against Myc (DSHB, AB_2266850) was performed to confirm proper expression of the MFN2 variant. Mitochondrial morphology was scored by analysis of mito-DsRed as described previously [10] . Cells were imaged with a Plan NeoFluar ×63 objective on a Zeiss 410 laser scanning confocal microscope (Carl Zeiss MicroImaging, Inc.). Analytical ultracentrifugation Twenty micromoles of MFN1 IM and MFN2 IM mixed with 1 mM GDP, 1 mM BeSO 4 , and 10 mM NaF were applied to AUC in a buffer containing 20 mM Tris, pH 8.0, 150 mM KCl, and 5 mM MgCl 2 . Sedimentation velocity experiments were performed with an An-60 Ti rotor at a speed of 145,000 g in a ProteomeLab XL-I Protein Characterization System (Beckman Coulter) at 20 °C. All interference data were processed according to a c(s) distribution model. Spectroscopic tethering assay Purified MFN1 IM -TM, MFN2 IM -TM, and corresponding mutants were reconstituted into preformed liposomes (83.5:15:1.5 mol % POPC/DOPS/Rhodamine-DPPE) as previously described [33] . Two micromoles of protein was reconstituted into 2 mM liposome in buffer H (25 mM HEPES, pH 7.4, 150 mM KCl, 10% glycerol), and detergent was removed by Biobeads. Five millimoles of MgCl 2 was added immediately before measuring the absorbance at 405 nm. Data were collected every 30 s using a Microplate Reader (Tecan). The absorbance before nucleotide addition was set to zero. To verify reconstitution efficiency, 30 µl proteoliposomes were mixed with 100 µl of 1.9 M sucrose and overlaid with 100 µl of 1.25 M sucrose and 20 µl buffer H supplied with 1 mM EDTA and 2 mM β-ME. After centrifugation in a Beckman TLS-55 rotor at 174,000 g for 75 min at 4 °C, 50 µl fractions were collected from the top of the gradient. Top and bottom fractions were analyzed by SDS-PAGE. Visual tethering assay POPC, DOPS, Texas Red DHPE, or Oregon green 488 DHPE (ThermoFisher) were mixed in a molar ratio of 84.5:15:0.5 as previously described [51] . Overall, 0.3 μM MFN1 IM -Sac1 TM or MFN2 IM -Sac1 TM or corresponding mutants were reconstituted into 0.6 mM prepared liposomes with Texas Red DHPE or Oregon green 488 DHPE in a buffer containing 20 mM HEPES, pH 7.5, 150 mM NaCl, 5 mM KCl, 5% glycerol, and 2% β-ME. Proteoliposomes labeled with red and green dyes were 1:1 mixed, 1 mM ligands and 5 mM MgCl 2 were subsequently added. Samples were incubated at 37 °C for 0.5 h before imaged by a confocal laser scanning microscopy (OLYMPUS FV1000). Surface conservation plot Protein sequences of 24 mitofusins were aligned using Clustal Omega [60] ( https://www.ebi.ac.uk/Tools/msa/clustalo/ ). These sequences from 12 vertebrate species included MFN1 and MFN2 from Homo sapiens (UniProt accession Q8IWA4 and O95140, respectively), Sus scrofa (M3VH65 and F1RF76), Bos taurus (F1MPL1 and D7GLD0), Equus caballus (F6VTU8 and F6YL70), Ovis aries (W5QHQ0 and W5Q8M0), Canis lupus familiaris (F1Q1G1 and E2R3M9), Oryctolagus cuniculus (G1SEC8 and G1SU75), Felis catus (A0A1D5PYU0 and M3VU19), Mus musculus (Q811U4 and Q80U63), Gallus gallus (A0A1D5PER5 and E1BSH7), Xenopus tropicalis (Q28FR9 and F6QKB9), and Danio rerio (Q6PFP9 and A8WIN6), The alignment result and structure of MFN2 IM -GDP complex were uploaded to the ConSurf online server [61] ( http://conseq.tau.ac.il ) to compute conservation scores for the residues. Surface plot of MFN2 IM with conservation score-based coloring was generated using PyMOL Molecular Graphic Systems (version 0.99, Schröinger LLC; http://www.pymol.org/ ). Pull-down assay Twenty micrograms of GST-tagged MFN1 IM was incubated with 60 μg MFN2 IM with or without 2 mM corresponding ligand for 2 h at 4 °C in a buffer containing 20 mM HEPES, pH 7.5, 150 mM NaCl, 5 mM MgCl 2 , and 1 mM DTT. 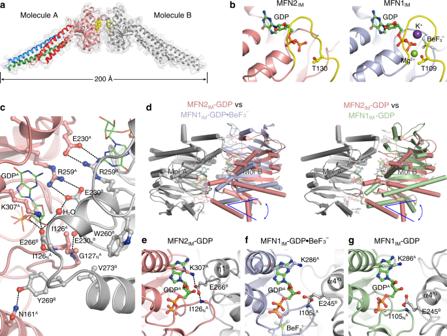Fig. 3 Dimerization of MFN2IMvia the G domain.aThe MFN2IMdimer in GDP-bound state, with transparent surface representation. Molecule A is colored as in Fig.1b, molecule B is in gray. GDP is shown as yellow spheres.b, Switch I configuration of MFN2IM-GDP structure and MFN1IM(Protein Data Bank code 5YEW) in the transition state. Switch I is colored yellow. The catalytic residues MFN2IM(Thr130) and MFN1IM(Thr109) are shown as ball-and-stick models.cDetails of the G interface of MFN2IM. Only one side of the G interface is shown for other involved residues except for the central dual salt bridges.dStructural comparison of MFN2IM-GDP dimer with MFN1IM-\({\mathrm{GDP}} \bullet {\mathrm{BeF}}_{3}^{-}\)dimer (PDB code 5YEW, left) and with MFN1IM-GDP dimer (PDB code 5GOM, right). The structures are superimposed for one polypeptide chain (Mol A, shown in gray). The positions of the other chain (Mol B) showed a clear difference in orientation between MFN2IM(pink) and MFN1IMstructures (light blue or green). Comparison of the G interface of MFN2IMin the GDP-bound state (e) between MFN1IMin the transition state (fPDB code 5YEW) and in the GDP-bound state (gPDB code 5GOM). Note the MFN2-specific Glu266-Lys307 salt bridge and the tighter trans association The mixtures were sampled to 100 μg GST beads (GE Healthcare) and then washed with the same buffer. Proteins retained by the GST beads were eluted by extra 20 mM GSH before analyzed by SDS-PAGE. Native PAGE Blue native PAGE technique was used to check the homo- and hetero-dimerization of MFN2 IM . Ten micromoles of MBP-tagged MFN1 IM /MFN2 IM was mixed with 10 μΜ untagged MFN1 IM /MFN2 IM in the absence or presence of tenfold concentration of indicated nucleotides for 2 h at room temperature. The samples were then mixed with 5× loading buffer (1%[w/v] bromophenol blue, 50%[v/v] glycerol) and subjected to native PAGE analysis at 4 °C. 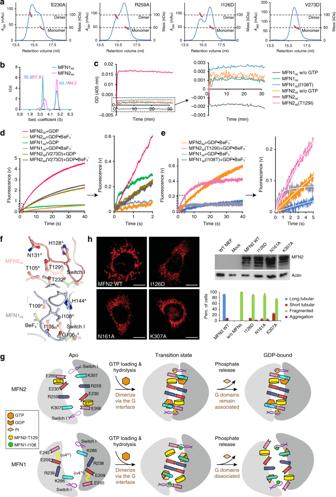Fig. 4 Characterization of MFN2IMdimeric interface.aDimerization property of the G interface mutants in the presence of\({\mathrm{GDP}} \bullet {\mathrm{BeF}}_{3}^{-}\)was assayed by analytical gel filtration coupled to RALS. Calculated molecular masses at the absorption peaks of 280 nm are plotted in red. mAU milli-absorption units.bAUC results of MFN2IMand MFN1IM(theoretical molecular mass 52.6 and 50.9 kDa, respectively) in the presence of\({\mathrm{GDP}} \bullet {\mathrm{BeF}}_{3}^{-}\). The estimated molecular masses determined by sedimentation velocity are given in kilodaltons (kDa) above the peaks.cLiposome tethering assay for wild-type MFN2IM-TM/MFN1IM-TM and mutants. A representative plot from three independent experiments is shown.dDimerization via the G interface slows down the nucleotide exchange of MFN2IMand MFN1IM. The initial part of each fluorescence trace was magnified.eEffect of MFN2IM(T129I) and MFN1IM(I108T) on the nucleotide exchange efficiency in the dimeric state. The initial part of each fluorescence trace was magnified and fitted to exponential function as shown in a white curve.fSurroundings of MFN2-Thr129 and MFN1-Ile108 in the dimerization form.gModel for comparison between MFN2 and MFN1 in G domain dimerization. Note the tighter G interface of MFN2 and its sustained dimerization in the GDP-bound state. Pi denotes phosphate group.hMitochondrial elongation assay with quantification for wild-type MFN2 and G interface mutants. Representative images are shown.Mfn1/2-null MEFs were transduced with retrovirus expressing 16× Myc-tagged WT Mfn2 or G interface mutants. Actin was used as a loading control. A lysate from WT MEFs is shown for comparison. For each construct, 100 cells were scored in biological triplicate. Error bars indicate s.e.m. Scale bars, 10 μm. Source data are provided as a Source Data file Electrophoresis was performed at 100 V for 20 min in 4% stacking gel, and then 160 V for 70 min in separating gel. The gel was stained with Coomasie brilliant blue. FRET assay MFN1 IM (C156S + A696C), MFN2 IM (C390S + A706C), and related mutants were labeled with fivefold concentration of fluorescent dye Cy3 or Cy5 (GE Healthcare) for 60 min at 4 °C in a buffer containing (20 mM HEPES, pH 7.5, 150 mM KCl, 5 mM MgCl 2 , and 0.5 mM Tris(2-carboxyethyl)phosphine (TCEP). Free dye was removed by gel filtration chromatography using a Superdex 200 10/30 column. Cy3 was excited at 537 nm, with peak emission at 570 nm. Cy5 fluorescence emission was detected at 667 nm. 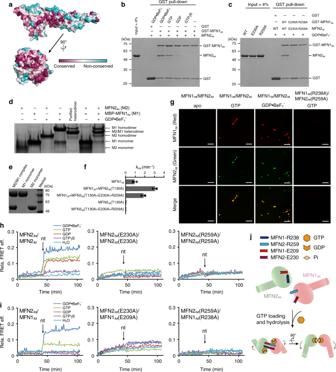Fig. 5 MFN2 interacts with MFN1 via G domain.aSurface conservation analysis reveals that the G interface is a highly conserved area in mitofusins.bPull-down assays showing the interaction between MFN2IMand GST-tagged MFN1IMin different nucleotide-loading conditions.cPull-down assays showing that the interaction between MFN2IMand MFN1IMis dependent on the G interface.dNative PAGE result showing the association between MFN2IMand MBP-fused MFN1IM.eSDS-PAGE showing the purified MFN2IM/MBP-MFN1IMhetero-complex.fMFN2IMstimulates GTP turnover of MFN1IM. Overall, 0.25 μM MFN1IMand 2.5 μM MFN1IMMFN2IMmutants were used.gLiposome tethering assay for wild-type MFN2IM/MFN1IMand G interface mutants. Representative images from five independent experiments are shown. Scale bar, 50 μm.hFRET experiment showing the G domain dimerization-dependent conformational change of MFN2IMin different nucleotide-loading conditions. The time point for the addition of corresponding nucleotides is indicated by an arrow for each panel. nt denotes nucleotide.iFRET experiment showing the conformational change of MFN2IMand MFN1IMupon association via the G domains in GTP- and\({\mathrm{GDP}} \bullet {\mathrm{BeF}}_{3}^{-}\)loading conditions.jA model for thetransassociation between MFN2IMand MFN1IM. Source data are provided as a Source Data file Cy3- and Cy5-labeled proteins (1 μΜ each) were mixed in a buffer containing 20 mM HEPES, pH 7.5, 150 mM KCl, 5 mM MgCl 2 , and 2% β-ME as previously described [33] . Fluorescence was measured once every 1 min in a flat black 96-well plate for 40 min, then 2 mM indicated nucleotide was added and the measurement continued for another 60 min. FRET traces were calculated as: FRET = I Cy5 /( I Cy3 + I Cy5 ), where I Cy3 and I Cy5 are the instantaneous Cy3 and Cy5 fluorescence intensities, respectively. Circular dichroism Proteins were diluted to 0.1 mg ml −1 in ddH 2 O and applied to CD measurements using a Chirascan spectrometer (Applied Photophysics) in quartz cuvettes with path length of 0.5 mm. Spectra were recorded from 180 to 260 nm at a bandwidth of 1 nm. 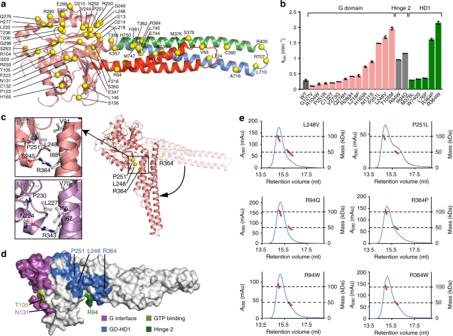Fig. 6 Characterization of CMT2A-related mutants.aOverview of the CMT2A-mutation sites on MFN2. The CMT2A-related single-point mutation sites are specified as yellow spheres on MFN2IMstructure colored as in Fig.1b.bGTP turnover rates of selected CMT2A-related MFN2IMmutants in comparison with wild-type MFN2IM. Locations of these mutants are color-specified.cCMT2A-mutation sites on the putative G domain-HD1 contact of MFN2 in the transition state. The structural model of rearranged MFN2IMis generated base on the MFN1IM-\({\mathrm{GDP}} \bullet {\mathrm{BeF}}_{3}^{-}\)structure (PDB code 5YEW). CMT2A-related residues and their potential interaction partners are presented as ball-and-stick models.dFunctional zones of MFN2 and the involved CMT2A-mutation sites.eDimerization property of CMT2A-mutants on the putative G domain-HD1 interface in the presence of\({\mathrm{GDP}} \bullet {\mathrm{BeF}}_{3}^{-}\). Source data are provided as a Source Data file 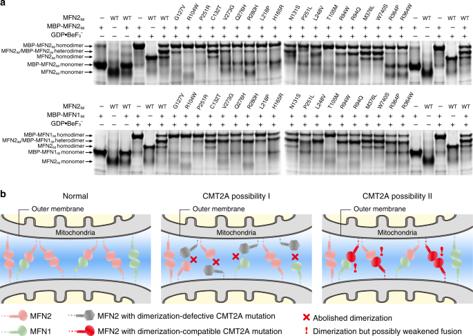Fig. 7 Interaction between CMT2A-related mutants and wild-type MFN1/2IM.aG domain-mediated association of CMT2A-related MFN2IMmutants with MBP-fused MFN2IM(upper) or MBP-MFN1IM(lower) tested by native PAGE.bSchematic drawing showing the two causes of CMT2A onset that may be derived from different MFN2 mutations. Source data are provided as a Source Data file All data were collected using a stop resolution of 1 nm and time per point of 0.5 s. A control spectrum obtained from the diluted buffer was subtracted from the original data. CD readouts were converted to mean residue ellipticity (M.R.E). Reporting summary Further information on research design is available in the Nature Research Reporting Summary linked to this article.